Quantum yield and excitation rate of single molecules close to metallic nanostructures The interaction of dyes and metallic nanostructures strongly affects the fluorescence and can lead to significant fluorescence enhancement at plasmonic hot spots, but also to quenching. Here we present a method to distinguish the individual contributions to the changes of the excitation, radiative and non-radiative rate and use this information to determine the quantum yields for single molecules. The method is validated by precisely placing single fluorescent dyes with respect to gold nanoparticles as well as with respect to the excitation polarization using DNA origami nanostructures. Following validation, measurements in zeromode waveguides reveal that suppression of the radiative rate and enhancement of the non-radiative rate lead to a reduced quantum yield. Because the method exploits the intrinsic blinking of dyes, it can generally be applied to fluorescence measurements in arbitrary nanophotonic environments. Understanding and quantifying the interaction between fluorescent dyes and metallic structures is vital for the design and development of nanophotonic applications, for example, for the fields of nanoapertures [1] or fluorescence enhancement [2] , [3] , [4] . Fluorescence enhancement, for example, has tremendous potential for biosensing, nanoscale light control and single-molecule applications, while nanoapertures (zeromode waveguides (ZMWs)) have already been commercially used for third generation DNA sequencing [5] . The fluorescence of a dye molecule is a function of the properties of the dye and its interaction with the environment. Modification of the environment by dielectric interfaces [6] , [7] , microresonators [8] , photonic crystals [9] , or metallic nanostructures [10] , [11] , [12] , [13] , [14] can alter the local electric field, which directly affects the excitation rate k ex (ref. 15 ), as well as influence the emission properties, namely the quantum yield Ф and even the angular emission pattern [16] . Together, this can result in fluorescence quenching [17] or enhancement [2] , [3] , [4] , depending strongly on the geometry and the orientation with respect to the excitation polarization [18] . Hence, understanding and quantifying the interplay between dyes and metallic nanostructures is a requisite to control fluorescence emission at the nanoscale and to exploit it for various applications. The excitation process can be reduced to the determination of the local electric field intensity either analytically for certain geometries [11] , [19] or solving Maxwell’s equations using FDTD simulation software [20] . The emission process is altered because the nanostructure can mediate the emission affecting the radiative decay rate k r by modifying the available radiative decay channels [21] . In addition, non-radiative decay channels k nr are also altered by energy transfer to dark modes of the metallic nanostructure [10] . These processes have been theoretically studied following the work by Gersten and Nitzan [22] , [23] , [24] , [25] , [26] and by numerical simulations [2] , [27] . Despite these developments, numerical and theoretical predictions could barely be contrasted with experimental measurements. On the one hand, it is difficult to produce nanophotonic structures with a defined position of a dye molecule [3] , [28] , [29] . On the other hand, there is no reliable experimental method to disentangle the three unknown rates in Φ (defined as k r /( k r + k nr )) and k ex from the typical parameters measured in single-molecule experiments, the fluorescence intensity and fluorescence lifetime. While there are some examples of single-molecule quantum yield measurements, they rely on sophisticated experimental design which is not easily accessible including, for example, photothermal imaging to measure the absorption cross-section [30] , or the detailed knowledge of a system and its precise electric field distribution [18] . Other methods require detailed knowledge of the optical mode density and cannot be applied to arbitrary objects [31] . A different approach by Wenger et al . [32] , [33] determined all relevant rates using fluorescence saturation but had to average over an ensemble of molecules sacrificing spatial resolution. The rates determined by this approach are additionally sensitive to higher excited state processes such as reverse inter-system crossing [34] . In this work, we use the blinking kinetics of a single fluorescent dye as third parameter besides intensity and fluorescence lifetime to determine the three characteristic rates k ex , k r and k nr for single dye molecules next to metallic structures. To test the method, we employ DNA origami structures [35] that enable accurate spacing and orientation of a dye and a 20 nm gold nanoparticle (NP) with respect to each other and with respect to the excitation light [3] , [17] . For validation, we use an over-determined system in which k ex is not enhanced because the dye is placed below the NP and compare our data to expectations from numerical simulations. We then place dye molecules in more complex environments such as next to larger metallic NPs and in small nanoapertures in thin metal films, so-called ZMWs. ZMWs are a key technology in single-molecule real-time sequencing [5] because they enable single-molecule measurements at higher, biologically relevant concentration [36] . However, the influence of the nanophotonic environment on the fluorescence of dyes immobilized in these nanoapertures has not yet been well-characterized. Our data determined with dyes in ZMWs of different diameters reveal the distributions of the localization-dependent properties within the ZMWs as well as a size-dependence of individual rate changes. Photophysical model and derivation of the analysis method We describe the photophysics of a fluorescent dye as a three level system ( Fig. 1a ): the electronic ground state S 0 , the first excited singlet state S 1 and a triplet state T 1 . We consider the excitation rate k ex for the S 0 – S 1 transition and the rates of de-excitation S 1 – S 0 via radiative and non-radiative processes k r and k nr , respectively. All these rates are altered in the proximity of plasmonic structures. However, since the presence of these plasmonic structures does not alter the spin–orbit coupling, the intrinsic inter-system crossing rate k ISC , which defines the S 1 - T 1 transition, remains constant [7] . 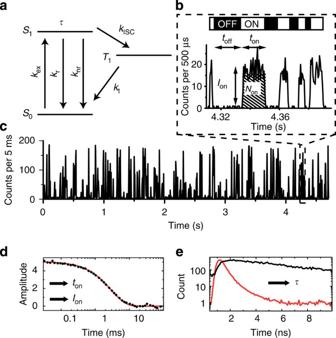Figure 1: Transition rates and experimental observables. (a) Jablonski diagram with relevant states and transition rates. (b,c) Fluorescence transient of an Atto647N dye molecule (500 μM ascorbic acid, enzymatic oxygen removal) at 0.5 and 5 ms binning, illustrating the observablesIon,tonandNon. (d,e) The corresponding autocorrelation function and fluorescence decay exhibit monoexponential behaviour and are used to extractIon,tonandτ. The red lines represent a monoexponential fit to the data (d) and the instrument response function (e). Figure 1: Transition rates and experimental observables. ( a ) Jablonski diagram with relevant states and transition rates. ( b , c ) Fluorescence transient of an Atto647N dye molecule (500 μM ascorbic acid, enzymatic oxygen removal) at 0.5 and 5 ms binning, illustrating the observables I on , t on and N on . ( d , e ) The corresponding autocorrelation function and fluorescence decay exhibit monoexponential behaviour and are used to extract I on , t on and τ . The red lines represent a monoexponential fit to the data ( d ) and the instrument response function ( e ). Full size image During the time the fluorescent dye performs cycles between S 0 and S 1 , termed t on ( Fig. 1b,c ), the molecule is bright. This cycling can be interrupted when a transition to the triplet state T 1 occurs with a probability given by k ISC /( k r + k nr +k ISC ). From fluorescence transients of single molecules and their fluorescence lifetime histograms we obtain the three experimental observables, the time before inter-system crossing occurs, t on , the intensity during the on-state I on ( Fig. 1b ) and the fluorescence lifetime τ ( Fig. 1e ). At non-saturating conditions, I on and t on are determined by autocorrelation analysis also using the mean intensity ( Fig. 1d ) (for details see Methods and Supplementary Note 1 ). The average time spent in a certain state is given by the inverse of the sum of all rates depopulating that state [37] , hence t off =1/ k t with the total triplet decay rate k t , and t on (see Fig. 1a,b ) can be expressed as [38] : which represents the product of the average time spent in S 0 before absorbing a photon, 1/ k ex , and the average number of cycles before a transition to T 1 occurs, ( k r + k nr + k ISC ) /k ISC , with the fluorescence lifetime τ =( k r + k nr + k ISC ) −1 . The fluorescence intensity is defined as I on = k ex k r τη = k ex Φη (refs 10 , 39 ) where η is the collection efficiency of the experimental set-up and Φ = k r τ represents the fluorescence quantum yield. These expressions are valid away from saturation where k ex ≪ (k r + k nr + k ISC ) and therefore τ ≪ 1/ k ex . In the following, primed variables (′) indicate the situation in presence of a plasmonic structure. Compared with k r and k nr , the rate of inter-system crossing k ISC is small and is therefore omitted in the lifetime definition τ =1/( k nr + k r ). From equation (1), the inverse of k ISC is eliminated to obtain k ex t on τ = k ′ ex t ′ on τ ′. With this, the change in excitation rate is determined based on changes in the fluorescence lifetime and the on-time: From comparing the intensities with and without the nanostructure and using equation (2), we obtain the change of the radiative rate: Here, α = η / η represents the change in collection efficiency. For the presented NP measurements, we assume constant collection efficiency η′ = η ( α =1), while the ZMW geometry is discussed in more detail below. Finally, the relative changes of quantum yield and of the non-radiative rate are determined from the initial quantum yield Φ and equation (5): Distance-dependent quenching of fluorescence To test our method, we design a series of fluorescent dye-NP systems, for which no significant excitation enhancement is expected. This is achieved by attaching a dye molecule in a plane below the gold NP, whereas electric field enhancement is expected in the equatorial plane of the NP (ref. 17 ) when illuminated from below ( Fig. 2a , for more details see Supplementary Table 1 ). 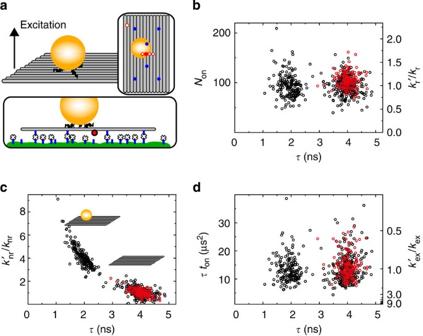Figure 2: Dye-NP arrangement using DNA origami and photophysical rate determination from single molecules. (a) sketch of the rectangular DNA origami attached to the coverslip via BSA/biotin/neutravidin/biotin bonds (lower inset) and positions of the gold NP (yellow, 20 nm diameter), biotin modifications (blue) and all five possible positions of the dye Atto647N (red; right inset) (b–d) Single-molecule photophysical rates for the sample with largest dye-NP distance (27.8 nm, red circles,n=140) and for the second closest distance of 8.3 nm (black circles,n=475). For the shorter distance, a population with reduced fluorescence lifetime is revealed that indicates the presence of a NP. Whilekr(b) andkex(d) are not altered,knris significantly increased (c). Changes of rate constants are normalized to the mean value of the population without NP. Figure 2: Dye-NP arrangement using DNA origami and photophysical rate determination from single molecules. ( a ) sketch of the rectangular DNA origami attached to the coverslip via BSA/biotin/neutravidin/biotin bonds (lower inset) and positions of the gold NP (yellow, 20 nm diameter), biotin modifications (blue) and all five possible positions of the dye Atto647N (red; right inset) ( b – d ) Single-molecule photophysical rates for the sample with largest dye-NP distance (27.8 nm, red circles, n =140) and for the second closest distance of 8.3 nm (black circles, n =475). For the shorter distance, a population with reduced fluorescence lifetime is revealed that indicates the presence of a NP. While k r ( b ) and k ex ( d ) are not altered, k nr is significantly increased ( c ). Changes of rate constants are normalized to the mean value of the population without NP. Full size image A rectangular DNA origami is attached to the surface ( Fig. 2a ). The dye Atto647N is attached to a staple strand below the DNA origami, whereas a 20 nm DNA functionalized gold NP is bound to the top of the DNA origami via hybridization in unzip geometry [40] for capturing strands protruding from the top of the DNA origami ( Fig. 2a ). We used five different DNA origamis varying the position of the fluorescent dye relative to the NP surface in the distance range of 6.6–27.8 nm (assuming a distance of 0.34 and 2.7 nm between two adjacent base pairs and two adjacent helices, respectively [35] , [41] , [42] ; for detailed DNA origami sequences see Supplementary Fig. 1 and Supplementary Table 1 ). The distance between the NP and the DNA origami surface is estimated by taking the average of sterically hindered full hybridization and a minimum stable hybridization of 15 bp from all three capturing strands. Practically, we expect a narrow spread for the dye-NP distance because we see no broadening of the lifetime distribution for constructs with NP ( Fig. 2b–d ) [17] . The assembly of the DNA nanostructures is controlled by atomic force microscopy (AFM) ( Supplementary Fig. 2 and Methods ) and sample immobilization is carried out according to ref. 17 , for details see Methods. Single-molecule measurements are carried out with a confocal microscope using a 640 nm pulsed laser diode for excitation. After scanning an area, identified molecules are placed in the laser focus and fluorescence transients are recorded. We use 500 μM ascorbic acid and remove oxygen in the measurement buffer to reduce every transient triplet state to a radical anion state, leading to longer off-times in the transient that are directly observable [43] , [44] . The method can be carried out with triplet states directly as demonstrated below for the ZMWs, but redox blinking improves visualization ( Fig. 1b,c ). Results are equivalent for 100% yield of reduction from the triplet state because the length of the off-states is irrelevant for analysis. For the DNA origami with the largest distance of 27.8 nm, we observe no difference of the fluorescence lifetime of 4.0 ns compared with a DNA origami sample without particle ( Fig. 2b–d , red data points). In contrast, for a fluorescent dye at a distance of 8.3 nm to the NP surface we observe two populations ( Fig. 2b–d , black data points). The population that coincides with the population at 4.0 ns is assigned to DNA origamis without NP and the population at 1.9 ns represents DNA origamis carrying a NP (for exemplary fluorescence transients see Supplementary Fig. 3 ). We now apply our data analysis to extract the changes of the respective rates relative to the rates in the absence of the NP using equations (2), (5), (6) and (7). The data in Fig. 2b reveal that for the distance of 8.3 nm there is no obvious change of the radiative rate constant k r , whereas the non-radiative rate constant k nr is significantly enhanced ( Fig. 2c ). The excitation rate constant is essentially unchanged ( Fig. 2d ), supporting our assumption that the excitation is not strongly affected when the dye is placed below the plane of the NP. We therefore measure three parameters to calculate essentially only two unknown variables so that the system is over-determined. This allows evaluating our method by calculating the same variables using different independent observables. If the excitation rate is unchanged, the quantum yield can, for example, be calculated from the fluorescence intensity [12] ( Φ ′ /Φ = I ′ on /I on ) or, using our method, from the fluorescence lifetime and the number of photons detected during an on-state (equation (6)). Both methods provide identical values for the quantum yield and also for the individual rate constants k nr and k r ( Supplementary Fig. 4 ). This substantiates our method and the underlying assumptions of, for example, an unchanged inter-system crossing rate constant k ISC . The comparison of experimental results with FDTD simulations is shown in Fig. 3a–d (refer to the Methods section for simulation details). As all measurements are carried out in aqueous solution with free rotation of the dyes around the linkers, the experimental values are expected to lie in between the values simulated for the two extreme orientations of the dipole, tangential or radial to the NP surface. In the radial orientation, the dye can couple more efficiently to the NP, which results in a shorter fluorescence lifetime compared with the tangential orientation. Any averaging is only an approximation, but the expected tendency is a gradual shift from a geometric weighting (2 × tan:1 × rad) at long fluorescence lifetimes towards a higher weighting of the radial component when the lifetime is in the range of the rotational correlation time of the dye, that is, in the order of 100 ps (ref. 3 ). 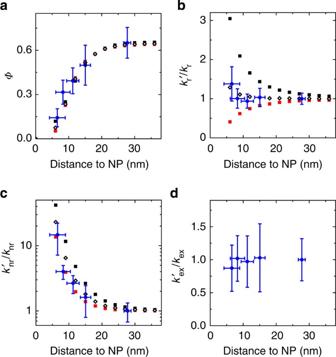Figure 3: Distance-dependent changes of the photophysical properties. (a) Distance dependence of the fluorescence quantum yield (blue, error bars indicate distance range from possible degree of hybridization and s.d. of the distribution resulting from equation (6)). Simulated values are shown for the radial orientation of the dye transition dipole moment with respect to the NP surface (black), as well as for the perpendicular orientation (red) and geometric averaging (hollow diamonds). (b–d) Distance dependence of photophysical rate changes forkr(b, mean+s.d. ofNon′/Nondistribution, see equation (5) andFig. 2b),knr(c, calculated from equation (7) with mean+s.d. ofτ′/τandNon′/Non) andkex(d, mean+s.d. of distribution from equation (2), seeFig. 2d). Sample size:n=140, 181, 59 and 147 for dyes at a distance ofd1=6.6 nm,d2=8.3 nm,d3=11.2 nm andd4=15.0 nm from a 20 nm NP; andn=197, 294, 103 and 129 for the reference molecules without NP. At distance ofd5=27.8 nm, no influence of the NP can be observed (n=140). The experiment was replicated three times. Figure 3: Distance-dependent changes of the photophysical properties. ( a ) Distance dependence of the fluorescence quantum yield (blue, error bars indicate distance range from possible degree of hybridization and s.d. of the distribution resulting from equation (6)). Simulated values are shown for the radial orientation of the dye transition dipole moment with respect to the NP surface (black), as well as for the perpendicular orientation (red) and geometric averaging (hollow diamonds). ( b – d ) Distance dependence of photophysical rate changes for k r ( b , mean+s.d. of N on ′/ N on distribution, see equation (5) and Fig. 2b ), k nr ( c , calculated from equation (7) with mean+s.d. of τ ′/ τ and N on ′/ N on ) and k ex ( d , mean+s.d. of distribution from equation (2), see Fig. 2d ). Sample size: n =140, 181, 59 and 147 for dyes at a distance of d 1 =6.6 nm, d 2 =8.3 nm, d 3 =11.2 nm and d 4 =15.0 nm from a 20 nm NP; and n =197, 294, 103 and 129 for the reference molecules without NP. At distance of d 5 =27.8 nm, no influence of the NP can be observed ( n =140). The experiment was replicated three times. Full size image The quantum yield ( Fig. 3a ) exhibits the expected distance dependence with quenching at close proximity of dye and NP. The experimentally determined rate constants for radiative and non-radiative transitions, which are the variables that define the emission process, are also well-described by the simulations ( Fig. 3b,c ). While the change of k r is small for 20 nm particles, even the expected increase for the shortest distance is reflected. We observe changes of the non-radiative rate by more than one order of magnitude that dominates the fluorescence lifetime at shorter distances. The excitation rate remains constant ( Fig. 3d ) in accordance with the previously mentioned expectation that no fluorescence enhancement occurs for a dye below the NP. Rate enhancement for different NP sizes In the next step, we employ a DNA nanopillar, consisting of a 12-helix bundle with a broader base. We can position the dye molecule in the equatorial plane of a gold NP with respect to the direction of the excitation light. This design has been used to enhance the fluorescence with one or two NPs of various sizes [3] , [18] (for the structure see Supplementary Fig. 5 ), and we in fact see that radiative, non-radiative and excitation rate are enhanced while the quantum yield is reduced for a dye positioned 11.5 nm away from a 20 nm gold NP ( Fig. 4 ). With increasing particle size (40 and 80 nm) all of these properties increase, but the quantum yield is in all cases reduced compared with the intrinsic quantum yield of Atto647N ( Fig. 4 ). 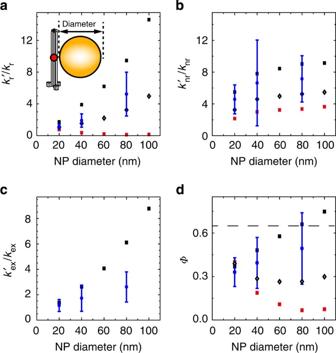Figure 4: Particle size-dependent changes of the photophysical properties for single molecules positioned at the equatorial plane. (a–c) Changes of the rate constantskr(a),knr(b) andkex. (c). In this configuration (sketch ina, for more details seeSupplementary Fig. 5and refs3,45), all relevant photophysical rates are enhanced with increasing particle size. Ina,b, simulated values are shown for the radial orientation of the dye transition dipole moment with respect to the NP surface (black), as well as for the perpendicular orientation (red) and geometric averaging (hollow diamonds). Inc, the simulated change in the excitation rate was averaged over all possible orientations to consider circularly polarized light. (d) The quantum yield also increases with the NP size, but is generally lower than the intrinsic quantum yield of Atto647N, indicated by a dashed black line. Error bars are represented as mean+s.d. of the values calculated for all molecules. Sample size:n=148, 142 and 69 for NPs of 20, 40 and 80 nm diameter, respectively; andn=214, 226 and 154 for the reference molecules without NP. The experiment was replicated three times. Figure 4: Particle size-dependent changes of the photophysical properties for single molecules positioned at the equatorial plane. ( a – c ) Changes of the rate constants k r ( a ), k nr ( b ) and k ex . ( c ). In this configuration (sketch in a , for more details see Supplementary Fig. 5 and refs 3 , 45 ), all relevant photophysical rates are enhanced with increasing particle size. In a , b , simulated values are shown for the radial orientation of the dye transition dipole moment with respect to the NP surface (black), as well as for the perpendicular orientation (red) and geometric averaging (hollow diamonds). In c , the simulated change in the excitation rate was averaged over all possible orientations to consider circularly polarized light. ( d ) The quantum yield also increases with the NP size, but is generally lower than the intrinsic quantum yield of Atto647N, indicated by a dashed black line. Error bars are represented as mean+s.d. of the values calculated for all molecules. Sample size: n =148, 142 and 69 for NPs of 20, 40 and 80 nm diameter, respectively; and n =214, 226 and 154 for the reference molecules without NP. The experiment was replicated three times. Full size image The resulting fluorescence intensity is changed by a factor of 0.58, 1.17 and 2.95, which is in agreement with previously published values [3] . To evaluate the contribution of the individual rates to these opposing effects from quenching to enhancement, we used our method for rate determination and compared the results to FDTD simulations. We observe that the changes in radiative and non-radiative rate are generally matching the FDTD simulations within experimental error ( Fig. 4a,b ). Furthermore, the notion that for stronger coupling of the dye to the NP the radiative rate exceeds the rate expected from geometric averaging is well-reflected. The instrument response function (IRF) of our setup is substantially broader (FWHM=600 ps) than the fluorescence lifetime of some of the brighter molecules (see Supplementary Fig. 5 for exemplary decay) so that for 13% of the molecules of the 80 nm sample we are not able to accurately determine the fluorescence lifetimes. These molecules are therefore ignored for analysis where the fluorescence lifetime is used leading to a slight underestimation of the excitation rate. This can, however, not explain why the excitation rate is generally lower than that expected from simulations ( Fig. 4c , see Supplementary Fig. 6 for electric field distribution around the NPs). A bias of our analysis method can be excluded because variation of the excitation intensity by more than one order of magnitude can be adequately detected ( Supplementary Fig. 7 ). The effect can partly be explained by the use of a high numerical aperture (NA) objective that leads to a superposition of various angles of incidence, yielding a smaller field enhancement than that expected from simulations that assume an incident plane wave acting on the NP. The lower excitation rate enhancement can also be related to a substantial orientational distribution of the DNA nanopillar with respect to the surface that has recently been characterized by three-dimensional super-resolution microscopy [45] . This orientational distribution only contributes to a broadening of k ex , whereas other factors increasing heterogeneity, such as the particle size and NP-dye distance, would also alter k r and k nr . Since we do not observe a clear correlation of the radiative rate change with the change of the excitation rate within a population (see Fig. 5 ), we conclude that heterogeneity is predominately induced by the orientational distribution of the DNA origami structures on the surface. 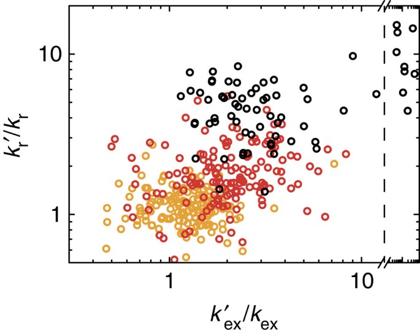Figure 5: Correlation of radiative and excitation rate with particle size. Radiative versus excitation rate constants of molecules with gold NPs of different sizes (20 nm: gold,n=148; 40 nm: red,n=142; 80 nm: black,n=69) normalized to the mean value of the molecules without NP for each particle size (for comparison to reference molecules seeSupplementary Fig. 8). The data points for one particle size do not exhibit a strong correlation between excitation and radiative rate constant. Data points beyond the break are not considered for the excitation rate because their fluorescence lifetime could not be determined accurately due to the temporal resolution of our experimental set-up. Figure 5: Correlation of radiative and excitation rate with particle size. Radiative versus excitation rate constants of molecules with gold NPs of different sizes (20 nm: gold, n =148; 40 nm: red, n =142; 80 nm: black, n =69) normalized to the mean value of the molecules without NP for each particle size (for comparison to reference molecules see Supplementary Fig. 8 ). The data points for one particle size do not exhibit a strong correlation between excitation and radiative rate constant. Data points beyond the break are not considered for the excitation rate because their fluorescence lifetime could not be determined accurately due to the temporal resolution of our experimental set-up. Full size image Rate suppression in ZMWs Next, we study the interaction of fluorescent dyes with a very different nanophotonic system. We immobilize single molecules in ZMWs of different sizes [46] . Light cannot propagate through these nanoapertures of subwavelength dimension in metal films, and evanescent excitation is restricted to a small volume close to the glass bottom of the ZMWs. Single dye molecules are immobilized via DNA origami nanodisks (63.6 nm diameter, see Supplementary Fig. 9 for AFM image; and ref. 47 for immobilization strategy) with one Atto647N dye located on the top side and four biotins on the bottom side in ZMWs (Pacific Biosciences, see Supplementary Fig. 10 for SEM images) of different sizes [46] . The nanodisk binds to the neutravidin-modified glass bottom of the ZMWs ( Fig. 6a,b ). This prevents direct contact of the dye with the metal and glass surfaces of the ZMW although we position the dye close to the edge of the nanostructure to probe all possible dye positions ( Fig. 6a–c ). When small molecules like DNA strands are randomly deposited in a ZMW, the radial distribution is simply proportional to the square of the distance from the centre, as it depends on the available surface at a given distance. For larger structures like the DNA nanodisk with a dye located off-centre, this distribution is not trivial and we obtain the radial distribution of distances d between dye and the ZMW wall from simulations of possible positions and orientations of the DNA nanodisk ( Fig. 6c , for details see Methods section). 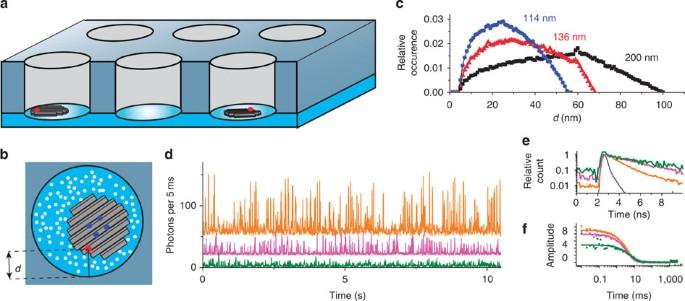Figure 6: Single-molecule fluorescence in ZMWs. (a) Sketch of the DNA nanodisks with the fluorescent dye Atto647N (red circle) immobilized in ZMWs (b) top view of one ZMW: the fluorophore is located close to the edge of the DNA nanostructure on the upper side to explore the whole aperture area without direct contact to the metal or the surface. Possible binding sites (neutravidin, white) are randomly distributed on the ZMW surface, but four biotins on the lower centre (positions indicated in blue) control the binding position and orientation. (c) Distance distribution between the dye and the ZMW wall from 100,000 simulated nanodisks for aperture diameters of 114 nm (blue circles), 136 nm (red triangles) and 200 nm (black squares). See Method section for details. (d) Fluorescence transients of three individual molecules in 114 nm ZMWs reveal the heterogeneity that arises from the random positioning of the dye. Molecule 1: orange, offset 50/(5 ms), molecule 2: magenta, offset 20/(5 ms), molecule 3: olive, no offset. (e) Corresponding fluorescence lifetime decays (black:IRF) (f) Corresponding AC functions. Figure 6: Single-molecule fluorescence in ZMWs. ( a ) Sketch of the DNA nanodisks with the fluorescent dye Atto647N (red circle) immobilized in ZMWs ( b ) top view of one ZMW: the fluorophore is located close to the edge of the DNA nanostructure on the upper side to explore the whole aperture area without direct contact to the metal or the surface. Possible binding sites (neutravidin, white) are randomly distributed on the ZMW surface, but four biotins on the lower centre (positions indicated in blue) control the binding position and orientation. ( c ) Distance distribution between the dye and the ZMW wall from 100,000 simulated nanodisks for aperture diameters of 114 nm (blue circles), 136 nm (red triangles) and 200 nm (black squares). See Method section for details. ( d ) Fluorescence transients of three individual molecules in 114 nm ZMWs reveal the heterogeneity that arises from the random positioning of the dye. Molecule 1: orange, offset 50/(5 ms), molecule 2: magenta, offset 20/(5 ms), molecule 3: olive, no offset. ( e ) Corresponding fluorescence lifetime decays (black:IRF) ( f ) Corresponding AC functions. Full size image The three exemplary fluorescence transients depicted in Fig. 6d illustrate the variety of behaviours obtained with molecules in ZMWs of 114 nm diameter. For these measurements, we enzymatically remove oxygen to induce triplet blinking that causes a monoexponential decay of the autocorrelation functions ( Fig. 6f ). Since the high off-time/on-time ratio together with scattering from the metal structure leads to pronounced scattering background in the fluorescence lifetime decay, we limit the lifetime analysis to photons during on-times (see Supplementary Figs 11 and 12 for photon selection and background correction). The brightest molecule (orange) has a shorter lifetime ( Fig. 6e ) than a molecule of medium intensity (magenta) or a dim molecule (olive), yet all molecules are darker than reference molecules on glass. This is in accordance with results from recent measurements in identical ZMW samples, where the fluorescence of all dyes was quenched [47] , whereas other studies have reported either quenching or enhancement [48] , [49] , [50] , [51] , [52] , [53] , [54] . The difference is likely related to the coating of the ZMWs used for specific immobilization, which keeps the molecules from the edges and the glass bottom. With classical analysis of intensity and fluorescence lifetime, there are multiple interpretations that can explain a reduced lifetime and intensity, based on the interplay between reductions or enhancements of the excitation rate and the quantum yield. Simulations of the electric field enhancement are not sufficient to resolve this because the position of the individual molecule in the ZMWs is unknown. With our analysis of blinking kinetics, however, we can disentangle the individual response of each molecule to the ZMW. 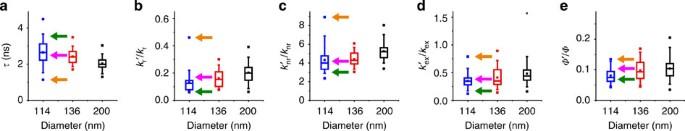Figure 7: Change of photophysical properties in nanoapertures of different diameters. (a) Fluorescence lifetime distribution of single dye molecules in ZMWs of 114, 136 and 200 nm diameter (n=45, 45 and 90, respectively). The points indicate maximum, mean and minimal value, the whiskers and box include 95–5% and 75–25%, respectively, and a horizontal line at the median value of the distribution. Orange, magenta and green arrows point to the properties of the three selected molecules fromFig. 6. Thex-axis is not to scale for better readability. (b–e) Distributions for change in radiative (b), non-radiative (c) and excitation rate (d) as well as changes of the quantum yield (e). A general trend to lower photophysical rates and quantum yields and consequently longer fluorescence lifetimes is observed when the aperture diameter is reduced. The experiment was replicated two times. Figure 7 presents the distributions of the fluorescence lifetime, the change of the radiative, non-radiative and excitation rate, as well as the change of the quantum yield for single molecules in ZMWs of 114, 136 and 200 nm diameter, respectively (see Fig. 7a–e ). For the analysis, the relative collection efficiency α =0.73 was used assuming that the emission into the buffer is completely suppressed (for details see Supplementary Fig. 13 ). While different values for α influence the absolute rate changes slightly, they do not affect the observed trends between ZMW diameters as is shown in Supplementary Fig. 14 , where we additionally calculated the results for the extreme cases of identical collection efficiencies ( α =1) and 100% collection efficiency with the ZMW sample ( α =0.54). The results of the molecules in Fig. 6d are indicated by the orange, magenta and olive arrows. Figure 7: Change of photophysical properties in nanoapertures of different diameters. ( a ) Fluorescence lifetime distribution of single dye molecules in ZMWs of 114, 136 and 200 nm diameter ( n =45, 45 and 90, respectively). The points indicate maximum, mean and minimal value, the whiskers and box include 95–5% and 75–25%, respectively, and a horizontal line at the median value of the distribution. Orange, magenta and green arrows point to the properties of the three selected molecules from Fig. 6 . The x -axis is not to scale for better readability. ( b – e ) Distributions for change in radiative ( b ), non-radiative ( c ) and excitation rate ( d ) as well as changes of the quantum yield ( e ). A general trend to lower photophysical rates and quantum yields and consequently longer fluorescence lifetimes is observed when the aperture diameter is reduced. The experiment was replicated two times. Full size image While the non-radiative rate is in all cases the only rate that experiences enhancement, both radiative and excitation rate are reduced compared with measurements outside the ZMWs. The reduction of the excitation rate for all diameters ( Fig. 7d ) can be explained by the evanescent nature of the excitation field [1] , an intrinsic property of the ZMW, and considering that our nanostructure positions the dye ~15 nm above the ZMW bottom. There is, however, a broad distribution of excitation rates due to the heterogeneous electric field distribution within the ZMW in accordance with simulations [1] , [51] , [55] . Furthermore, the excitation rate is stronger reduced for smaller ZMW diameters ( Fig. 7d ; ref. 1 ). From a reciprocity point of view this also explains why the radiative rate is stronger reduced in smaller apertures ( Fig. 7b ; ref. 56 ). Notably, this correlation between excitation and radiative rates cannot be explained with artifacts from our analysis, since the excitation rate is inversely proportional to the measured on-time and fluorescence lifetime, while the radiative rate is proportional to the on-time. The probably most surprising finding is that the fluorescence lifetime increases with decreasing aperture diameter [47] ( Fig. 7a ). This comes along with smaller non-radiative rate enhancement of small apertures compared with larger apertures ( Fig. 7c ) and is counterintuitive considering the distance distribution between the dyes and the ZMW metal surface. For the smaller apertures, the dyes are on average closer to the ZMW wall than for the larger apertures ( Fig. 6c ) and proximity to metal is generally associated with strongly distance-dependent quenching via non-radiative decay pathways (ohmic losses). This is also reflected within each sample, as the highest electric field intensity (and highest excitation rate) is expected close to the walls of the ZMW and the molecules with highest excitation rate also tend to have the highest radiative and non-radiative rate (see Supplementary Fig. 15 for correlations of the 114 nm sample). In summary, we present a simple method to determine the individual contributions of excitation, radiative and non-radiative rate changes that are typical for the interaction of dyes and nanophotonic structures. We demonstrate our analysis for both triplet and redox blinking of organic dyes. Single molecules are used as ultimately small probes to report on the electromagnetic environment in the near-field of self-assembled DNA-metal nanostructures and in ZMWs. For evaluating the method, we placed dyes at well-defined positions with respect to NPs and the excitation light on rectangular DNA origamis. With one 20 nm Au particle, we observe the expected distance-dependent quenching of intensity and fluorescence lifetime for dyes located outside the plane of excitation enhancement, which is dominated by changes of the non-radiative rate. When placing dyes in the equatorial plane of gold NPs of varying size, we observe an increase of the three relevant rate constants and an inhomogeneous broadening that we mainly ascribe to the orientational distribution with respect to the excitation light. In case of commercially used ZMWs, we find a correlation between excitation and emission rates for Atto647N molecules immobilized via DNA nanodisks. However, both excitation and radiative rates are suppressed and result in a lower fluorescence than from molecules outside a ZMW. In addition, we find that against intuition the fluorescence lifetime is longer and the non-radiative rate is smaller in smaller ZMWs although the dye is on average positioned closer to the metal. The method should be generally applicable to all sorts of photonic structures, such as micro-resonators, photonic crystals, ZMWs, interfaces, nanoantennas and other nanostructures without the need for modifications of common single-molecule set-ups. Sample preparation for DNA origamis with NPs NPs are functionalized with a T 15 -DNA strand with a thiol modification on the 5′-end according to ref. 57 . The DNA origami structures are folded as described previously [35] . For details on the nanostructures see Supplementary Table 1 (rectangular DNA origami) and refs 3 , 45 (DNA nanopillar). The DNA origamis are filtered three times with a buffer containing 1 × TAE and 12.5 mM MgCl 2 (Amicon Ultra-0.5 ml Centrifugal Filters, 100,000 MWCO, Millipore) at 14,000 r.c.f. for 8 min and then recovered for 2 min at 1,000 r.c.f. Attachment of the gold NPs is carried out after immobilization of the DNA origamis to avoid aggregation and to control the labelling yield. The DNA origamis are immobilized on BSA/BSA–biotin/neutravidin surfaces as shown in ref. 58 in 1 × PBS with 12.5 mM MgCl 2 . After the DNA origamis are bound we incubate the sample with a buffer containing 1 × PBS, 700 mM NaCl (+12.5 mM MgCl 2 for the nanopillar measurements) and the gold NPs of the different sizes until roughly half of the DNA origamis is equipped with a NP, while the other half serves as an internal reference at the exact same measurement conditions. The final measurement buffer consists of 1 × PBS, 12.5 mM MgCl 2 , 500 μM ascorbic acid, 1% (w/w) glucose and 10% (v/v) of an enzymatic oxygen scavenging system (30% (v/v) glycerol, 1 mg ml −1 glucose oxidase, 50 μg ml −1 catalase, 12.5 mM KCl and 0.1 mM Tris(2-carboxyethyl) phosphinehydrochloride in 50 mM TRIS pH 7.5). Sample preparation DNA nanodisk and ZMWs For details on the nanodisk structure see Supplementary Table 2 . Folding was carried out over 3 days (for folding programme see Supplementary Table 3 ) in 1 × TAE buffer containing 12.5 mM MgCl 2 . The DNA origamis are filtered three times at 15,000 r.c.f. for 5 min (Amicon Ultra-0.5 ml Centrifugal Filters, 100,000 MWCO, Millipore) with pH 7.4 MOPS buffer containing 50 mM MOPS, 75 mM potassium acetate and 12.5 mM magnesium acetate. The sample is recovered for 3 min at 3,000 r.c.f. We purchase ZMW samples from Pacific Biosciences, where the ZMW chip is mounted on a conventional microscope slide. Each chip provides six different ZMW diameters ranging from 85–200 nm. The glass bottom of the ZMW chip is already functionalized with PEG–biotin to allow immobilization of neutravidin-labelled molecules [46] . The chip is washed twice with MOPS buffer before incubation with 1 mg ml −1 neutravidin in MOPS buffer. After five more washing steps, the DNA origami sample is added and the binding process is controlled by confocal imaging. Once a reasonable occupancy is reached, the sample is thoroughly washed to remove unbound DNA structures. Measurements are carried out in MOPS buffer with 1% (w/v) glucose and 10% (v/v) of the oxygen scavenging system. AFM imaging AFM imaging is performed in solution on a NanoWizard 3 ultra AFM (JPK Instruments AG, Berlin, Germany) in TAE buffer (40 mM TRIS, 2 mM EDTA and 12.5 mM MgCl 2 ). Therefore a freshly cleaved mica surface (Quality V1, Plano GmbH, Wetzlar, Germany) is incubated with a 10 mM NiCl 2 solution for 2 min, rinsed with milliQ water and air dried . The surface is incubated for 2–5 min with diluted DNA sample (1 μl for rectangular origami or 2 μl for nanodisc in 10 μl TAE buffer). After that the surface is washed five times with TAE buffer to remove unbound DNA samples. For image analysis, we use the JPK Data Processing Software (JPK Instruments AG). Single-molecule fluorescence microscope Single-molecule fluorescence transients are measured with a custom built confocal set-up based on an inverted microscope (IX71, Olympus) with a high NA oil immersion objective (× 60, NA 1.35, UPLSAPO 60XO for rectangular DNA origami; × 100/NA 1.40, UPLSAPO100XO for DNA nanopillar and ZMWs, both Olympus). The ATTO647N dye molecules are excited at 640 nm with an 80 MHz pulsed laser diode (LDH-D-C-640, Picoquant, 2.5 μW for rectangular DNA origami, 1.5 μW for DNA nanopillar measurements, 5 μW for ZMW measurements). A combination of linear polarizer and quarter wave plate ensures circular polarization of the laser beam, which is guided to the sample by a dichroic beamsplitter (Dualband z532/633, AHF). The surface with immobilized DNA origamis is imaged by scanning the sample with a piezo stage (P-517.3CL, Physik Instrumente). From that image, molecules are selected and placed in the laser focus for time resolved analysis. The resulting fluorescence is collected by the same objective and separated from the excitation light after focusing on a 50 μm pinhole by two filters (Bandpass ET 700/75 m, AHF; RazorEdge LP 647, Semrock). The signal is detected by a single photon counting module ( τ -SPAD 100, Picoquant) and a PC-card for time-correlated single-photon counting (SPC-830, Becker&Hickl). The raw data is processed with custom made software (LabView2009, National Instruments). Autocorrelation analysis For autocorrelation analysis, we calculate the background corrected autocorrelation function after removing the constant offset of 1 The brackets denote temporal averaging, I(t) is the signal from one molecule and B is the background intensity. This results in an exponential decay which is fitted with The amplitude and decay time allows extraction of the on- and off-times With this information, the on-counts N on and the intensity during the on-state can be calculated: For a more detailed derivation of this analysis, see Supplementary Note 1 . Fluorescence lifetime analysis The fluorescence lifetime decay is deconvoluted with the IRF (shown, for example, in Fig. 1e ) using the commercial reconvolution software FluoFit (Picoquant). The software fits a convolution of an exponential decay with the IRF plus a multiple of the IRF as scattering contribution to the experimental lifetime decay. For this, a time independent background of the IRF and the experimental decay are considered as well as a shift of the decay with respect to the IRF. The fitting function stems from the FluoFit software information. Numerical simulations Numerical simulations were performed using commercial FDFD software ( www.cst.com ). The relative change in the excitation rate was estimated by simulating the electric field intensity in the vicinity of the NP system at the fluorophore position and averaged to consider a circular polarization. The relative change of the radiative and non-radiative rates were estimated following ref. 27 , where the dye is modelled by a dipole current source with a determined orientation. The total power radiated into the far field and dissipated by the metallic objects is computed and normalized to the total power radiated into the far field in the absence of metallic objects. For these calculations, the intrinsic quantum yield of the Atto647N dye of 0.65 was considered according to ref. 56 . All simulations were performed assuming a planar illumination with water as medium, mimicking the buffer conditions and effects arising from the glass/water interface were neglected. Simulations of dye distribution in ZMWs Considering the constant ZMW diameter of d ZMW , the nanodisk diameter d ND and the distance between the dye molecule and the centre of the DNA nanodisk d off , we simulate the position and orientation of the nanodisk. The distance between the nanodisk centre and the ZMW centre r is randomly chosen from the range [0, ( d ZMW − d ND )/2] with a normalized probability density function of p( r )~ r . Together with the angle θ chosen with equal probability from the range [0, 2 π ], this defines the position of the nanodisk in polar coordinates. In the same manner the rotation angle ψ of the nanodisk is simulated. With this, the distance d between dye and ZMW wall can be calculated as follows: How to cite this article: Holzmeister, P. et al . Quantum yield and excitation rate of single molecules close to metallic nanostructures. Nat. Commun. 5:5356 doi: 10.1038/ncomms6356 (2014).